Persistent super-diffusive motion ofEscherichia colichromosomal loci The physical nature of the bacterial chromosome has important implications for its function. Using high-resolution dynamic tracking, we observe the existence of rare but ubiquitous ‘rapid movements’ of chromosomal loci exhibiting near-ballistic dynamics. This suggests that these movements are either driven by an active machinery or part of stress-relaxation mechanisms. Comparison with a null physical model for subdiffusive chromosomal dynamics shows that rapid movements are excursions from a basal subdiffusive dynamics, likely due to driven and/or stress-relaxation motion. Additionally, rapid movements are in some cases coupled with known transitions of chromosomal segregation. They do not co-occur strictly with replication, their frequency varies with growth condition and chromosomal coordinate, and they show a preference for longitudinal motion. These findings support an emerging picture of the bacterial chromosome as off-equilibrium active matter and help developing a correct physical model of its in vivo dynamic structure. Chromosomal structure and dynamics in bacteria comprises a number of complex entangled phenomena, which has consequently led to a far more primitive understanding of its underlying physical characteristics in comparison to its eukaryotic counterpart [1] , [2] , [3] . Much of the complexity is a consequence of the lack of spatial compartments within the cell and a poorly characterized hierarchy in spatiotemporal dynamics throughout the cell cycle. For instance, short-timescale chromosome motion is likely dominated by the viscoelastic nature of the crowded cytosol–chromosome ensemble, but physical details of this complex medium are still poorly understood. At short timescales, when the contribution of segregation dynamics is negligible, individual loci ‘sub-diffuse’, that is, explore space with a shallower power law in time compared with Brownian motion. This behaviour is characterized by a robust scaling law for the mean-square displacement of a locus, specifically a power law in time with exponent α ≃ 0.4, consistent across many experimental conditions and chromosomal positions [4] , [5] , [6] . Similar scaling laws have been found for chromosomal loci in eukaryotes such as yeast [7] and humans [8] . Notably, the power law exponent ~0.4 is not reproduced by standard polymer models [6] . The cytosol is a highly crowded environment, which promotes the chromosome to be (semi-)collapsed due to osmotic self-attraction [9] , [10] . However, in vivo the compacted chromosome (nucleoid) maintains a well-defined shape and tends to occupy a significantly smaller volume than the cell, likely a result of the activity of numerous DNA-associated proteins with varying functionality [11] , [12] , [13] , [14] . The average mobility of loci is a function of chromosomal coordinate, suggesting spatially varying physical organization and/or noise levels due to transcription, translation or protein activity [4] . Furthermore, even at short timescales, non-equilibrium contributions are an essential component of chromosome dynamics. Recent work [5] has argued that ATP-dependent enzymatic activity generates non-thermal fluctuations of chromosomal loci that are larger than thermal fluctuations. These ‘active’ forces broadly categorize the nucleoid as an active material [15] . The physical organization of the nucleoid is dramatically rearranged on the timescale of the cell cycle, particularly during chromosome replication and segregation [2] . The sources of energy driving the segregation process are currently not clear. It is difficult to disentangle the process of segregation from the basal physical nature and organization of the nucleoid [3] . If segregation were a smooth process, it would appear as a drift over the underlying short-timescale subdiffusion. However, it has been reported that the spatial separation of sister chromosomes is not a continuous process but rather occurs as a small number of rapid chromosomal rearrangements [16] , [17] . This behaviour suggests the existence of energetic or entropic barriers for separation, likely in interplay with active force-generating processes. A recent imaging study [13] revealed further intriguing nucleoid density dynamics, measured by the dynamic intensity of a fluorescent fusion of the nucleoid-associated protein HU. Longitudinal ‘density waves’ appear to travel along the nucleoid, causing 5–10% density changes within 5 s. The same study found that sister chromosomes separate by a series of sequential discontinuous pulses, each elongating the nucleoid by 5–15%. The pulses appear to cluster at well-defined cell-cycle times. Here, we image fluorescently labelled chromosomal loci in E. coli across timescales of 0.1–100 s, and show that a significant number of locus trajectories contain a small but noticeable subset of abnormally elongated regions exhibiting significantly super-diffusive motion. These near-ballistic trajectories, which we term ‘rapid chromosomal movements’ (RCMs) are abnormal compared with sub-diffusion, and instead show a broad spectrum of velocities and a crossover from subdiffusive to ballistic dynamics. Rapid movements have a statistical tendency to be longitudinal and centrifugal, and their proportion increases in faster growth conditions. These results are consistent with the presence of nontrivial active/stress-release mechanisms, and support the physical picture of heterogeneous complex non-equilibrium motion superimposed on a viscoelastic background for the bacterial nucleoid. Persistent ballistic motion of chromosomal loci tracks We performed tracking measurements of the Ori2 and Ter3 loci strains, at 1-s frame separation. For each locus in a given medium we based our analysis on 3,000–7,000 tracks from five to nine different experiments. We noticed ( Fig. 1a ) that a small number of tracks (typically 50 to 350 of the 3,000 to 7,000 tracks analysed) were abnormally elongated and apparently directed (on the observation timescale). These trajectories occur in movies where, in the same field of view, most of the foci follow a subdiffusive motion, and there is no correlation between their occurrence in different cells, therefore discarding the possibility that they are artefacts caused by stage drift. To quantify these rare but atypical displacements, we considered, for single tracks, both time-averaged mean absolute displacements (MAD), defined as MAD( τ )=‹| x ( t + τ )− x ( t )|›, and time-averaged mean-squared displacements, MSD( τ )=‹( x ( t + τ )− x ( t )) 2 ›. For these elongated tracks, the MAD is linear in time (and the MSD quadratic) for all of the available time lags ( Fig. 1a,b ), indicating a directed displacement at constant velocity (up to 0.5 μm min −1 ). We also found a large number of tracks where this linear behaviour is visible in a smaller range of time lags. 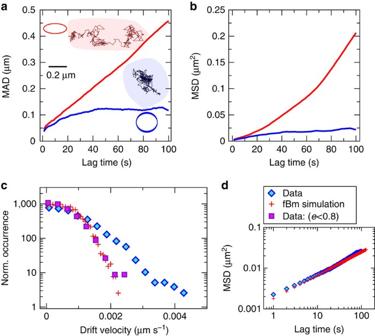Figure 1: Analysis of chromosomal loci trajectories. (a,b) Example comparing a ballistic (red) and a ‘typical’ (blue) track. The inertia ellipses of the two tracks are sketched next to them. The graphs are the time-averaged MAD (a) and mean square displacement (b) of the same two tracks, plotted as a function of time lag. (c,d) Ballistic tracks are statistically atypical. The point is shown by comparing the drift-velocity distribution with a parameter-matched fBm (c); experimental data (diamonds) have a much wider tail than simulated data (pluses). Restricting the data to tracks with low eccentricity (e<0.8, squares) restores the compatibility. Paneldshows that the ensemble-averaged MSD of the data and the simulations are nearly identical over the available timescales (error bars, s.e., are smaller than symbols, the parameters of the fBm are fixed by a fit of this curve, in this case MSD≃0.0019τ0.57μm2, the high exponentα=0.57 is caused by RCMs themselves, seeFig. 2and text). Data refer to the Ori2 locus for cells grown in minimal medium supplemented with CAA+Glu, imaged for 200 frames with frame separation of 1 s. Figure 1: Analysis of chromosomal loci trajectories. ( a , b ) Example comparing a ballistic (red) and a ‘typical’ (blue) track. The inertia ellipses of the two tracks are sketched next to them. The graphs are the time-averaged MAD ( a ) and mean square displacement ( b ) of the same two tracks, plotted as a function of time lag. ( c , d ) Ballistic tracks are statistically atypical. The point is shown by comparing the drift-velocity distribution with a parameter-matched fBm ( c ); experimental data (diamonds) have a much wider tail than simulated data (pluses). Restricting the data to tracks with low eccentricity ( e <0.8, squares) restores the compatibility. Panel d shows that the ensemble-averaged MSD of the data and the simulations are nearly identical over the available timescales (error bars, s.e., are smaller than symbols, the parameters of the fBm are fixed by a fit of this curve, in this case MSD ≃ 0.0019 τ 0.57 μm 2 , the high exponent α =0.57 is caused by RCMs themselves, see Fig. 2 and text). Data refer to the Ori2 locus for cells grown in minimal medium supplemented with CAA+Glu, imaged for 200 frames with frame separation of 1 s. Full size image This evidence suggests the presence of stages of rapid motion during the dynamics of loci, which take the form of super-diffusive transients, or of diffusion with a much larger mobility. These RCMs appear to intersperse the common basal subdiffusive dynamics found in the majority of tracks. We verified that images of segmented cells perfectly overlap before and after the measurement. Finally, in all experiments, RCMs are not observed in fixed cells, and thus cannot be dismissed as artefacts of image analysis. The deformation of each track can be quantified considering it as a cloud of points of unit mass, and computing its moment of inertia matrix with respect to the centre of mass [18] . Evaluation of the inertia ellipse of each measured track gives the major and minor axes (the eigenvectors of the inertia matrix), and an estimate for its elongation, given by its eccentricity e . We also defined an apparent ‘drift velocity’ v d as the vector between the first and the last point of the track, divided by the elapsed time. In presence of ballistic motion, the magnitude of this vector estimates its speed. The distribution over the tracks of υ d , the magnitude of v d projected on the main track axis, is plotted in Fig. 1c . This plot shows the existence of a continuous, wide spectrum of drift velocities, rather than a well-defined speed for the rapid movements. Comparison with fractional Brownian motion To test whether the observed rapid movements of a few tracks could be considered statistically relevant we considered subdiffusion, using the fractional Brownian motion (fBm) of ref. 19 as a null model. For each experimental condition, we simulated the same number of tracks and frames per track present in the experimental data. This theoretical description is minimal, in the sense that it can be fully constrained by the data: the two parameters of the simulation (Hurst exponent H = α /2, and apparent diffusion constant) were chosen by fitting the exponent and the prefactor of the MSD curve from experimental data ( Fig. 1d ). For all the analysed loci, we found that, at equal track-length, track sampling and number of tracks, the parameter-matched simulated data showed a considerably lower number of high- υ d tracks than the experimental ones, indicating that the phenomenon was significant ( Fig. 1c and Supplementary Fig. 1 ). The significance of a high- υ d track can be quantified by defining a P -value as the integral of the tail of the mahing fBm υ d distribution. For example, with this criterion, a track with υ d =0.0025 μm s −1 has P ≃ 5 × 10 −3 ( Supplementary Fig. 2 ). This analysis suggests a reasonable range for a cutoff in υ d to define the atypical tracks. We set this cutoff at P =5 × 10 −3 . With this choice, about 5% of the Ori2 tracks and 4% of the Ter3 tracks are identified as RCMs for growth at 30 °C on minimal medium supplemented with casamino acids and glucose, while for the same medium supplemented with glycerol ~2% of the tracks are identified as RCMs for both loci. Supplementary Figs 3 and 4 contain example tracks for RCMs defined with these criteria, for six loci analysed with 1-s frame separation. Note that in presence of pure subdiffusion, for example, for a fBm, υ d is just a measure of the apparent overall displacement of a short ‘walk’, and vanishes with increasing observation times. The comparison procedure just described quantifies the difference between an fBm expectation and the data at all timescales. Crossover between subdiffusive and ballistic behaviour The intertwining of basal subdiffusive motion and ballistic displacement limited to a few tracks is visible from sliding ensemble-averaged MAD curves ( Fig. 2a ). When restricted to trajectories with large υ d , these curves show a clear crossover from subdiffusive motion (with exponent α ≈0.4) to highly super-diffusive, near-ballistic behaviour. The crossover timescale is ~10 s. We also emphasize that the averaging is done by moving windows, so the motion is subdiffusive for short time lags throughout the whole trajectory. The fact that the rapid trajectories behave subdiffusively at short timescales suggests that these loci are not freed from the ‘mesh’ that gives rise to the subdiffusion. The same crossover is visible in the (sliding) ensemble-averaged MAD and MSD of all data, creating a noticeable upturn in these curves ( Figs 1d and 2a ). The upturn gradually disappears when the average is conditioned to the majority of tracks with small υ d ( Fig. 2a ). We also modelled this behaviour in terms of intermittency between two processes, estimating the subdiffusion from the tracks with low υ d and a ballistic motion from the tracks with high υ d ( Supplementary Fig. 5 ). 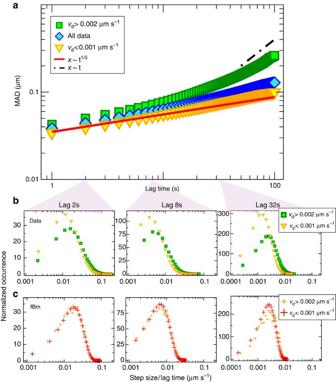Figure 2: Overlap between subdiffusive and directed motion. (a) Ensemble-averaged MAD (averages are performed with moving windows) versustrestricted to differentυdranges. For tracks withυd>0.002 μm s−1(squares), a clear crossover from subdiffusive (exponentH≈0.2) and ballistic motion is visible at a scale of ~10 s. Tracks withυd<0.001 μm s−1(triangles) almost completely comply with the subdiffusive law (these tracks comprise 70% of all tracks). The average of all tracks (diamonds) shows an upturn fort≳10 s, due to the outliers, compatible with the observed MSD exponentα≈0.57>0.4 (seeFig. 1d). (b) Distributions of step-size to lag time ratios at different timescales in experimental (top panel) and simulated (bottom panel) data. Tracks withυd>0.002 μm s−1(P=5 × 10−2, squares) show a shifted step-size distribution with respect to tracks withυd<0.001 μm s−1(triangles). For simulated data, this shift is absent at short lag time and only begins to appear at a lag time of 32 s. Data refer to the Ori2 locus for cells grown in minimal medium supplemented with CAA+Glu, imaged for 200 frames at 1-s intervals. Figure 2: Overlap between subdiffusive and directed motion. ( a ) Ensemble-averaged MAD (averages are performed with moving windows) versus t restricted to different υ d ranges. For tracks with υ d >0.002 μm s −1 (squares), a clear crossover from subdiffusive (exponent H ≈0.2) and ballistic motion is visible at a scale of ~10 s. Tracks with υ d <0.001 μm s −1 (triangles) almost completely comply with the subdiffusive law (these tracks comprise 70% of all tracks). The average of all tracks (diamonds) shows an upturn for t ≳ 10 s, due to the outliers, compatible with the observed MSD exponent α ≈0.57>0.4 (see Fig. 1d ). ( b ) Distributions of step-size to lag time ratios at different timescales in experimental (top panel) and simulated (bottom panel) data. Tracks with υ d >0.002 μm s −1 ( P =5 × 10 −2 , squares) show a shifted step-size distribution with respect to tracks with υ d <0.001 μm s −1 (triangles). For simulated data, this shift is absent at short lag time and only begins to appear at a lag time of 32 s. Data refer to the Ori2 locus for cells grown in minimal medium supplemented with CAA+Glu, imaged for 200 frames at 1-s intervals. Full size image However, the upturn in the MAD or MSD versus lag time plot (for lag times larger than ~10 s) persists when all data are averaged together. This explains why the fitted exponent α in the MSD plot in Fig. 1d , used to define the simulation, is larger than 0.4 (close to 0.6). The curve is a composition of short-time subdiffusive motion and faster motion on larger timescales. Using a fBm with the effective fitted exponent as a null model is a conservative choice, as it includes the (null) hypotheses that (i) the motion is purely subdiffusive and (ii) the displacement is closest to the experimental one for all the measured timescales. Conversely, an fBm with exponent α =0.4 fitting well the shorter timescales would underestimate the displacement at large timescales giving an even narrower distribution of expected υ d in the simulated data. The plots of the absolute displacement in Fig. 2a also show that the step-size is biased towards larger steps if tracks with increasingly larger υ d are included in the averages. To gain further insight into the properties of this mix of subdiffusive and ballistic motion, we analysed the distributions of the step-size to lag-time ratio, q ( τ )=| x ( t + τ )− x ( t )|/ τ , in experimental data and in parameter-matched fBm simulations ( Fig. 2b ). This ratio (dimensionally a velocity) quantifies the contribution of step-size to directed motion. The experimental data show a noticeable difference in the distributions conditional to high versus low υ d , while the same bias is nearly absent in the fBm simulations. At short timescales (<10 s), the slightly larger (on average) steps of RCMs do not increase in size when they are aligned with the main direction of the track; this bias is detectable only after time lags of ~10 s ( Supplementary Fig. 6 ). These trends in the step size might be used to define the tracks exhibiting rapid motion. The angular correlations show similar behaviour ( Supplementary Fig. 7 ). We quantified this by the angular correlation function , where is the unit vector directed as the step of time lag τ , x ( t + τ )− x ( t ). In this expression, we are fixing the elementary time step τ and then finding the angular correlation as a function of a lag δ . As expected from a fBm, for steps of short timescale, τ =1–2 s, the correlation function is negative for small δ , and relaxes to zero for increasing δ . This holds also for tracks with high υ d (both in experimental data and in simulations). For increasing τ , the angular correlation becomes positive with increasing δ , and this happens in both simulations and experimental data, with the crossover timescale being systematically smaller in experimental data. In brief, the rapid motions show a bias in both step size and angular correlations, but the bias in angular correlation is also observed in the (rarer) ‘extreme’ trajectories of a parameter-matched fBm, while the bias in step sizes seems more specific of the experimental data. Preferred direction and orientation of rapid movements To gain further insight on the features of RCMs, we analysed their direction and orientation ( Fig. 3 ). The orientation was measured as the smallest (0–90 degrees) angle from the main axis, keeping into account the mirror-flip cell symmetries. We found ( Fig. 3a ) that for the Ori2 locus, and for the Ter3 locus in the faster growth medium, there was a noticeable statistical tendency of RCMs to be more aligned with the cell’s long axis, while this tendency was lost for the Ter3 locus in slower growth conditions. Note that this trend is only statistical, and that many tracks with rapid movements have arbitrary orientations. The directionality was measured as the frequency of steps along the longitudinal cell axis in the outward versus inward directions with respect to the cell centre of mass. We found that the Ori2 locus had a noticeable bias for outwards rapid movements, while the same tendency was much weaker for normal trajectories ( Supplementary Fig. 8 ). By contrast, we did not find any strong correlation of the frequency of fast movements with particular initial or final subcellular localizations ( Supplementary Fig. 9 ). 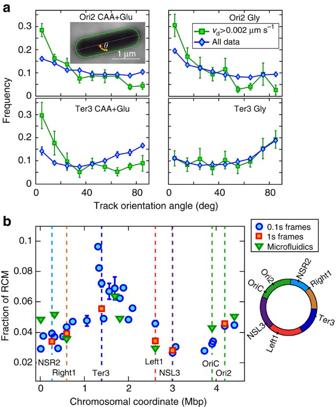Figure 3: Main biological properties of RCMs. (a) Orientation of the fast-moving trajectories (squares) compared with the general trends (diamonds), for Ori2 (top panels) and Ter3 (bottom panels) loci in cells grown at 30 °C in minimal medium supplemented with CAA and glucose (left panels) or with glycerol (right panels). With the exception of the Ter3 locus in slow-growing cells, there is a statistical trend of the rapid motions to be longitudinal (countering a global weakly transverse trend in the case of Ter3). Cells are imaged for 200 frames at 1 s frame separation. The angle is defined as illustrated in the inset, as the positive smallest angle between the main axis of the track and the longitudinal cell axis. Error bars (s.d.) are computed over biological replicates. (b) Fraction of rapid movements as a function of chromosomal coordinate. Squares correspond to the loci analysed in detail in this work, belonging to different macrodomains2as sketched in the right panel. The other symbols derive from experiments on 27 loci with frame separation of 0.1 s performed on agar pads4(circles) and in a microfluidics device (triangles)20. The cutoff for rapid movements is theP-valueP<5·10−3with respect to fBm null model matched with the mean behaviour of each locus separately (seeSupplementary Fig. 2). Cells are grown at 30 °C in minimal medium supplemented with CAA and glucose (seeSupplementary Fig. 10for other conditions). Figure 3: Main biological properties of RCMs. ( a ) Orientation of the fast-moving trajectories (squares) compared with the general trends (diamonds), for Ori2 (top panels) and Ter3 (bottom panels) loci in cells grown at 30 °C in minimal medium supplemented with CAA and glucose (left panels) or with glycerol (right panels). With the exception of the Ter3 locus in slow-growing cells, there is a statistical trend of the rapid motions to be longitudinal (countering a global weakly transverse trend in the case of Ter3). Cells are imaged for 200 frames at 1 s frame separation. The angle is defined as illustrated in the inset, as the positive smallest angle between the main axis of the track and the longitudinal cell axis. Error bars (s.d.) are computed over biological replicates. ( b ) Fraction of rapid movements as a function of chromosomal coordinate. Squares correspond to the loci analysed in detail in this work, belonging to different macrodomains [2] as sketched in the right panel. The other symbols derive from experiments on 27 loci with frame separation of 0.1 s performed on agar pads [4] (circles) and in a microfluidics device (triangles) [20] . The cutoff for rapid movements is the P -value P <5·10 −3 with respect to fBm null model matched with the mean behaviour of each locus separately (see Supplementary Fig. 2 ). Cells are grown at 30 °C in minimal medium supplemented with CAA and glucose (see Supplementary Fig. 10 for other conditions). Full size image RCM frequency varies with chromosomal coordinate We found that RCM frequency varies with chromosomal coordinate ( Fig. 3b ). The dependence of RCMs on chromosomal coordinate becomes weaker in slower growth conditions ( Supplementary Fig. 10 ). Additionally, we found a moderate trend relating RCMs to centripetal motion of Ter3 foci ( Supplementary Fig. 11 ). In faster growth conditions, the fraction of RCMs is anti-correlated with the variations in the apparent diffusion constant with chromosomal coordinate reported previously [4] . Rapid movements have a minor impact on the global apparent diffusion constant of loci, which is set by the great majority of subdiffusive tracks ( Supplementary Fig. 12 ). We also analysed a dataset of tracked chromosomal loci from Javer et al. [4] , extended with new experiments, in which typically ~450 images were taken at 0.1-s intervals. Here, typical values of υ d were larger by a factor of 2–4 than the values found in the tracks with 200 images taken at 1 frame per second (considering the first 100 frames in both data sets). This is likely connected to the fact that for an fBm, as previously discussed, the apparent υ d increases with decreasing observation time. Additionally, smaller distances are biased towards larger measured movements by increased photobleaching, because of larger uncertainty in the tracking, but also due to a possible decrease of the probe size [4] . While the biases due to probe size are hard to avoid, the measured offset suggests that, in order not to overestimate the fraction of RCMs, one reasonably needs to define a larger cutoff. Using fBm as a null model allows to determine this cutoff for each locus and timescale: the analysis presented in Fig. 1c (setting P =5 × 10 −3 ) was performed on each locus to score for atypical trajectories (obtaining cutoffs around υ d ≈0.006–0.008 μm s −1 for the 0.1 s frame separation data). With this procedure, experiments performed in microfluidic devices [20] and in agar pads at different timescales yield quantitatively consistent results, also indicating that the architecture and the flow of the observation chamber do not affect the measurements. RCMs and replication timing Notably, while the apparent diffusion constant of loci, and hence the subdiffusive contribution to their motion, does not seem to vary greatly across the tested (fairly slow) growth conditions, the fraction of RCMs seems to decrease coherently from richer to poorer growth media ( Fig. 4a ). In each medium, we asked whether cells with different numbers of optically resolved loci, and hence at different replication stages, produced differential fractions of rapid movements. However, the number of optically resolved loci is only weakly correlated with replication, since replicated loci can be catenated for 10 or more minutes [21] . Moreover, when multiple loci are observed, replication can be already finished ( Fig. 4b ). 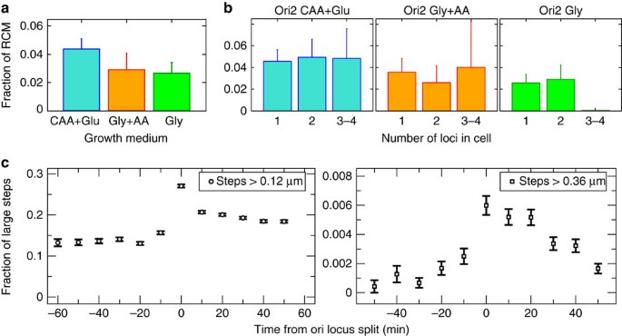Figure 4: RCMs and cell cycle. (a) Fraction of rapid loci movements in cells grown in different nutrient conditions (30 °C in minimal medium supplemented with casamino acids and glucose, amino acids and glycerol, or glycerol). Cells were imaged for 200 frames with frame separation of 1 s. Error bars refer to variations (s.d.) between different biological replicates (each with 1,000–2,000 imaged tracks). (b) Breakdown of the same data by number of optically resolved loci per cell (in slow growth conditions, rightmost panel, no cells with 3–4 foci are found). This index is a weak proxy for the stage in the replication cycle. (c) Fraction of 1-min steps with longitudinal projection longer than 0.12 μm (left) and 0.36 μm (right), plotted as a function of the segregation kinetics, for the OriC locus (982 tracks from two experiments). Cells were imaged and segmented every minute, in order to reconstruct the segregation cycle, and the data were synchronized by the time at which the replicated sister loci were resolved optically (origin of times in these plots). Data refer to AB1157E. coligrown at 30 °C in minimal medium supplemented with amino acids. Error bars (s.d.) are computed on the distribution of step sizes occuring at a given time. Figure 4: RCMs and cell cycle. ( a ) Fraction of rapid loci movements in cells grown in different nutrient conditions (30 °C in minimal medium supplemented with casamino acids and glucose, amino acids and glycerol, or glycerol). Cells were imaged for 200 frames with frame separation of 1 s. Error bars refer to variations (s.d.) between different biological replicates (each with 1,000–2,000 imaged tracks). ( b ) Breakdown of the same data by number of optically resolved loci per cell (in slow growth conditions, rightmost panel, no cells with 3–4 foci are found). This index is a weak proxy for the stage in the replication cycle. ( c ) Fraction of 1-min steps with longitudinal projection longer than 0.12 μm (left) and 0.36 μm (right), plotted as a function of the segregation kinetics, for the OriC locus (982 tracks from two experiments). Cells were imaged and segmented every minute, in order to reconstruct the segregation cycle, and the data were synchronized by the time at which the replicated sister loci were resolved optically (origin of times in these plots). Data refer to AB1157 E. coli grown at 30 °C in minimal medium supplemented with amino acids. Error bars (s.d.) are computed on the distribution of step sizes occuring at a given time. Full size image To achieve a better control on this question, we used data from experiments performed at a different timescale ( Fig. 4c ). Pictures of cells were taken at 1-min intervals, and the length of steps in the longitudinal coordinate for a locus close to Ori was recorded. In these experiments, the event of origin split, when the two sister origins are optically resolved, can be used as reference to align the trajectories, thereby achieving a better control on the segregation cycle. This allowed us to measure the fraction of longitudinal 1 min steps above a certain length cutoff as a function of time for ‘synchronized’ cells. This analysis was performed on ~1,000 tracks and a total of 150,000 steps. Owing to the practical difficulty in determining the exact splitting time in the synchronized trajectories we begin our analysis at the first time point where two distinct foci are observable. To avoid biases, we excluded the splitting event from the analysis, and considered only the large steps found more than 5 min before and after its occurrence. In this case, it was not possible to use fBm as a null model, because the displacement is dominated by directional biases [22] . Replication likely initiates 10–20 min before the splitting is observed [21] and proceeds for 40–50 min. We find that steps of medium-to-large size (above 0.12 μm, roughly comparable to the cutoff of υ d =0.002 μm s −1 used for RCMs) occur with noticeable frequencies well before the split event, indicating that they do not depend solely on replication (for example pre-replication large steps could be due to release from septum [23] , [24] ), Supplementary Fig. 13 . Only very large (and very rare) longitudinal steps (for example, above 0.36 μm in 1 min) appear to occur mainly after splitting (hence possibly co-occur with replication). We also considered similar data for the lac locus ( Supplementary Fig. 13 ), which show the same ubiquitous occurrence of steps above 0.12 μm (with an increase at splitting, and likely persisting after replication ends), together with 0.36 μm steps appearing only after splitting of the foci. Evidence across several experimental and biological conditions shows that RCMs are rare but significant. The strong points that enable our experiments to establish this are the abundance of data and the high time resolution. Quantitatively, fractions of RCMs may vary across experiments for several technical and biological reasons, but the different data sources are coherent once these factors are taken into account. Comparing data collected in the same conditions with different time resolutions (0.1 and 1 s time intervals), the distributions of measured υ d are different. However, a comparison with the null subdiffusion model leads to choose different υ d thresholds for the two kinds of experiments, which fully restores quantitative agreement in the fraction of RCMs between the data sets. Using the same criterion, the data are also consistent for different devices and conditions ( Fig. 3b and Supplementary Fig. 10 ). Finally, apparently larger and more frequent longitudinal long steps are found in the experiment with minute-scale time intervals and cell-cycle resolution. The quantitative differences likely lie in a technical offset, but one should also note that slightly different behaviour in nucleoid organization from strains MG1655 and AB1157 has been reported [25] , and might play a role here. Overall, despite of some technical intricacies, we conclude that our results are consistent across conditions, strains, laboratories and devices used to perform the experiment, indicating that the observed rapid chromosomal motions are not the product of artefacts. Similar long-range directed motions have also been reported in eukaryotes [26] , [27] . Our analysis does not allow to pinpoint a definite origin of these rapid motions. They can be connected to a set of different reported phenomena, some of which may be more or less frequent for different chromosomal regions, or even loci-specific. First, RCMs could be related to ‘snaps’ [13] , [16] associated with the segregation dynamics. For example, at the so-called ‘T2’ transition, one sister domain is reported to move half the length of the cell in a few minutes. In this case, a locus could be undergoing subdiffusive motion within a meshwork that, itself, is undergoing rapid directed motion due to a global rearrangement. Additionally, such global rearrangements are expected to also affect loci that are not within the main moving domains. Considering the average trajectories of the 1-min frame separation data, we did not find direct evidence of the discrete transitions in the cell cycle [13] , [16] , likely because our technique, compared with labelling of the whole chromosome, can only access a very limited spatial region at a time, the synchronization of the time series is imperfect, and averaging of a large number of tracks could ‘smooth out’ such effects. Also note that loci-specific splitting behaviour is expected. For example, the Ter3 locus is very close to the dif locus, which is involved in dimer reduction as well as in specific anchoring of its region to the cell septum, against the general tendency for the chromosome to be organized as a linear object [24] , [28] . We observe an RCM decrease when Ter3 is near the centre of the cell, and a mid-cell-oriented increase elsewhere ( Supplementary Fig. 11 ). Equally, Ori2 is within the domain that is affected by programmed release of oriC sisters [16] , [22] and ensuing replisome splitting, which occurs a few minutes later. The motions observed at Ori2 could reflect these effects. The null model tailored for each individual locus defined here assures that the RCM fraction is meaningful also in the presence of these biologically relevant heterogeneities. Second, it is interesting to compare our observations with another recent finding of Fisher et al. [13] : ‘density waves’ where a consistent fraction of the nucleoid mass is relocated in a few seconds. Some RCMs might be related to this phenomenon, since the crossover from subdiffusion to RCMs occurs around 10 s, in agreement with the timescale of 5 s emerging from the density waves and RCMs for some loci are consistent with a net average flow ( Fig. 3 and Supplementary Fig. 8 ). Third, RCMs could be related to the movement of decondensed nucleoid regions in time and space, which are generally reported in the literature. For example, ‘fingers’ of nucleoid material around the radial cell periphery with concomitant fluxes of density along its length were reported recently [13] . Decondensation rapid movements might explain the specificity of the Ter region ( Supplementary Fig. 8 ), which is reported to be more fluid and localized at the nucleoid periphery [29] , [30] (this happens far from cell divisions, when the Ter region is instead condensed and tethered [25] , [28] , [31] ). In the hypothesis of decondensation, loci that are freed from some chromosomal constraints might perform a faster random motion in the cytoplasm, but their trajectories could be persistent enough to be mistaken for near-ballistic at the observation timescale. This explanation cannot be generally applicable, as the average displacement would fail to show the crossover seen in Fig. 2 between short-time subdiffusion with exponent α ≃ 0.4 and near-ballistic motion at longer timescales. In other words, since even the RCMs are subdiffusive at short timescales, these loci are likely not locally freed from an underlying viscoelastic gel, as they would be if their motion were purely diffusive. On the contrary, the fact that many rapid movements are nearly ballistic (on the observation timescale) indicates that they are likely related to some active, possibly ATP-dependent process. As discussed in the introduction, ATP-dependent fluctuations of subdiffusive loci have been previously reported [5] , and interpreted as an ‘effective temperature’. We find that this description may be reductive, as RCMs span timescales that overlap with the subdiffusive motion. We surmise that an alternative physical picture could be a viscoelastic gel undergoing active mass-relocation or stress relaxation [32] . An effective-temperature description disregards this aspect. To test this, we performed a measurement 30 min after blocking ATP production, and found that, despite of a visible reduction in apparent diffusion, RCMs are still present ( Supplementary Fig. 14 ), confirming that relaxation of pre-stored stress might be in place (we speculate that measurements of two-loci short-time correlations could be useful to test this). This scenario could help resolving a puzzle raised by the results of Weber and co-workers [5] , [33] . In a gel, the amplitude of thermal fluctuations depends on the viscosity, which becomes time-dependent in presence of viscoelasticity. Weber and coworkers [5] , [33] reported that ATP depletion did not change the subdiffusive character of the motion, as the measured exponent α was ≃ 0.4 both before and after ATP depletion. In the framework of an effective temperature, this fact is surprising, since thermal driving forces and viscosity should be related, and led to suggest that the ATP-dependent fluctuations must have thermal-like time dependence to account for the lack of variation of the subdiffusive exponent upon ATP depletion. The properties of RCMs suggest that describing active motion purely as thermal-like fluctuations of non-thermal amplitude might be reductive. Such effects were first reported by Fisher and co-workers [13] , [16] , who, for example, observed that the splitting of the gln locus is accompanied by rapid, asymmetric separation of sister loci, indicating that the basis for the movement is accumulated stress within the nucleoid. More recently, they proposed that programmed intranucleoid ‘tethers’ (for example, by nucleoid-associated bridging proteins like H-NS or Fis, or by condensins like MukB), accumulate in inter-segment linkages, which, in combination with changes in supercoiling state, tend to put the chromosome in an unfavourable condition, promoting eventual catastrophic release of tethers. Release of entanglements (due to knots or unknotted states) by topoisomerases can also act in the same way. The same authors observe that pulses of longitudinal nucleoid elongation are preceded by nucleoid shortening (possibly due to a transient increase of bridging). An obvious candidate for the active accumulation of stress is genome replication, which, in a semi-compacted genome, likely generates nontrivial stress patterns by both adding new mass and affecting the supercoiling density, but these motions could also be generated by molecular motors (for example, the translocase FtsK is active during the late stages of cytokinesis and chromosome segregation, and the condensin ATP-ase MukB could perform some processive task), and by RNA polymerase itself, possibly through ‘transertion’ [34] , [35] (concurrent transcription and translation, leading to membrane localization of the genes encoding for membrane proteins). Note that some of these processes are expected to lead to many radial RCMs, in line with our observation that only a fraction of them are longitudinal. In our view, this stress-release dynamics makes the nucleoid unique with respect to other biological active gels that have been characterized [15] , [33] . In this scenario, active forces cause a build up of elastic stress, later released in intermittent cascades, similarly to off-equilibrium colloidal materials, and known biological gels [32] , [36] . This would also be consistent with the observed anti-correlation between apparent diffusion and RCMs ( Supplementary Figs 10 and 12 ), if we speculate that the constraints inhibiting subdiffusive mobility are the same as those that favour stress-releasing rapid motions. Strains and culture conditions To investigate chromosomal dynamics at short timescales, we used a collection of 27 E. coli strains derived from MG1655 with the GFP-ParB/ par S fluorescent label system (kindly provided by the Espéli and Boccard [17] laboratories). Two specific loci (Ori2 and Ter3) were selected for in-depth analysis. To explore the cell cycle dynamics at larger timescales, we used a derivative of AB1157 that incorporates both the the Fluorescent Repressor Operator System (FROS) and the ParB–parS system [22] . All the chemical reagents were obtained from Sigma-Aldrich unless otherwise stated. Strains were grown overnight in LB at 37 °C with ampicillin (100 μg ml −1 ). Cultures were diluted 200:1 into M9 minimal salts (Difco), supplemented with the following nutrients: (i) Casamino acids and glucose, CAA+Glu , doubling time 75 min; complementary salts (MgSO 4 2 mM, CaCl 2 100 μM, Tryptophan 4 μg ml −1 and thymidine 5 μg ml −1 ), 0.4% glucose and 0.5% casamino acids (Difco). (ii) Glycerol medium, Gly , doubling time 150 min, M9 minimal salts; complementary salts and 0.4% glycerol. (iii) Glycerol and amino acids, Gly+AA , doubling time 120 min; MgSO 4 2 mM, 0.2% glycerol, 100 μg ml −1 of each arginine, histidine, leucine, threonine, proline and 10 μg ml −1 thiamine hydrochloride. Cultures were grown at 30 °C to an OD 600 of 0.1–0.2 to reach early exponential phase. Microscopy For imaging at short times, 5 μl of the early exponential culture were deposited on a 1.5% agarose pad with the appropriate media. Details of the microscope setup are described elsewhere [4] . Two different protocols were used to acquire the short-time epifluorescence movies: movies of 450 frames with 0.1-s interval under continuous illumination, and movies of 200 frames with 1-s interval and 100 ms of illumination time per frame. A phase contrast image was recorded before and after the image stack acquisition. For the long-time experiments, phase contrast and fluorescence images were captured once per minute for 6–8 h, further details can be found in ref. 22 . Data analysis Experiments performed for this work (i) acquired new data at 1-s frame separation for 6 loci ( Supplementary Fig. 1 and Supplementary Table 1 ) and (ii) extended the 0.1-s frame separation dataset of Javer et al. [4] ( Supplementary Table 2 ), which was included in the analysis, together with data from ref. 20 (microfluidic chemostat). We added a total of 45 new experiments and 46,958 tracks to the analysis. Additionally, we used data from ref. 22 (long-time experiments), extended with 800 new trajectories and an experiment on the Lac locus. Movies were analysed with custom software written in MATLAB (Mathworks). The particle-tracking algorithm used to analyse the short- and long-time movies is presented in refs 4 , 22 . Cells were segmented from the phase-contrast images in order to express the foci trajectory in the cell coordinate system. How to cite this article: Javer, A. et al. Persistent super-diffusive motion of Escherichia coli chromosomal loci. Nat. Commun. 5:3854 doi: 10.1038/ncomms4854 (2014).